PYK2 sustains endosomal-derived receptor signalling and enhances epithelial-to-mesenchymal transition Epithelial-to-mesenchymal transition (EMT) is a central developmental process implicated in cancer metastasis. Here we show that the tyrosine kinase PYK2 enhances cell migration and invasion and potentiates EMT in human breast carcinoma. EMT inducer, such as EGF, induces rapid phosphorylation of PYK2 and its translocation to early endosomes where it co-localizes with EGFR and sustains its downstream signals. Furthermore, PYK2 enhances EGF-induced STAT3-phosphorylation, while phospho-STAT3 directly binds to PYK2 promoter and regulates PYK2 transcription. STAT3 and PYK2 also enhance c-Met expression, while c-Met augments their phosphorylation, suggesting a positive feedback loop between PYK2–STAT3–c-Met. We propose that PYK2 sustains endosomal-derived receptor signalling and participates in a positive feedback that links cell surface receptor(s) to transcription factor(s) activation, thereby prolonging signalling duration and potentiating EMT. Given the role of EMT in breast cancer metastasis, we also found a significant correlation between PYK2 expression, tumour grade and lymph node metastasis, thus, demonstrating the clinicopathological implication of our findings. Signal transduction cascades of cell surface receptors can induce diverse cellular responses in different cell types. The high diversity of signalling outcomes is largely dependent on the receptor type and its cognate ligand, and it is remarkably influenced by the duration of the signal [1] . Epidermal growth factor (EGF), for example, induces the transient activation of ERK1/2 in PC12 cells, and consequently triggers cell proliferation, whereas NGF induces persistent ERK activation and leads to cell differentiation [2] . Likewise, the transient activation of JNK promotes cell survival and proliferation, whereas prolonged JNK activation induces growth arrest and cell death [3] . Signalling duration can be controlled through both intracellular and extracellular mechanisms [4] . Internalization of cell surface receptors followed by receptor recycling to the cell surface prolongs receptor signalling, while routing the internalized receptors to lysosomal degradation terminates the signal [5] . This mechanism regulates the signalling duration of many growth factors receptors including EGF receptor (EGFR), c-Met [6] and transforming growth factor-β receptor (TGFβR) [7] and markedly affects cell fate. Positive and negative feedbacks are other key mechanisms that influence signalling duration and, consequently, switching cellular responses [8] . The switch in JNK from a transient to sustained activity, for example, is controlled by several positive feedback loops that lock JNK in a highly active state and promote cell death [9] . On the other hand, TMEPAI, a direct target gene of TGFβ signalling, desensitizes TGFβ signalling by interfering with Smad phosphorylation [10] . These examples demonstrate that the duration of the signal can be controlled at the level of the activated receptor, the accessibility of the ligand and by feedback loops between downstream pathways or effectors. Prolonged activation of transcription factors can also influence cellular response. Transient or sustained activation of NF-κB, for example, results in the expression of a distinct subset of target genes [11] . Similarly, sustained activation of c-Fos in mammary epithelial cells leads to epithelial-to-mesenchymal transition (EMT), characterized by the loss of cell polarity and increased invasiveness, whereas the transient activation of c-Fos in these cells results in a reversible loss of cell polarity [12] . EMT is a reversible multistep process defined by the loss of epithelial characteristics and the acquisition of a mesenchymal phenotype. This transition is accompanied by the disassembly of cell–cell contacts as well as by loss of cell polarity and E-cadherin expression, and by the acquisition of spindle-shaped morphology, high cell motility and invasiveness [13] , [14] , [15] . EMT can be triggered by various growth factors and cytokines including EGF, hepatocyte growth factor (HGF), fibroblast growth factor, TGFβ and bone morphogenetic proteins (BMP) as well as by the WNTs and Notch signalling pathways [16] , [17] . Yet, the functional acquisition of EMT and its long-term maintenance requires sustained activation of inducible signals. Transient exposure of mammary cells to TGFβ, for example, is sufficient to induce the characteristic morphological and molecular changes of EMT. These changes, however, are not sustained for long periods [18] , [19] . Maintenance of TGFβ-induced EMT requires a sustained signal, leading to activation of the transcription factor Twist1 and maintenance of late EMT response [19] . Hence, multiple cellular mechanisms control the signalling duration and thereby affect EMT initiation and its subsequent long-term maintenance. Here we show that the non-receptor tyrosine kinase PYK2 is functionally involved in EMT in human mammary cells. PYK2 is an important regulator of multiple signalling pathways that control cell growth, proliferation, survival, polarity, migration and invasion [20] , [21] , [22] , [23] . It mediates diverse signalling pathways of various cell surface receptors in a cell type-specific manner, and it is implicated in the tumorigenesis and metastasis of many human cancers [24] , [25] , [26] , [27] . Although previous studies suggest that PYK2 positively regulates EMT [23] , [28] , the mechanisms underlying its function in EMT have not been fully explored. Our studies suggest that PYK2 employs two major mechanisms to prolong EMT-associated signals. First, it sustains endosomal-derived receptor signalling and consequently postpones signal termination. Second, it participates in a positive feedback loop that links cell surface receptor(s) to transcription factor(s) activation, thereby persisting initial EMT signals and promoting late EMT response. Elevated PYK2 expression enhances EMT in mammary cells Previous studies have shown that TGFβ induces EMT in mammary breast cancer cells and concomitantly elevates the expression of PYK2 protein [28] . To better characterize the effects of EMT inducers on PYK2 expression, we assessed its protein level in MCF10A and MDA-MB-468 cells in response to two potent EMT inducers: TGFβ and EGF. The immortal mammary human epithelial MCF10A cells undergo EMT in response to EGF or TGFβ [29] , whereas MDA-MB-468 cells, an invasive human breast carcinoma, undergo EMT in response to EGF [30] . As shown in Fig. 1a , both EGF and TGFβ enhanced the expression of PYK2 in MCF10A cells as well as of fibronectin and vimentin, two mesenchymal markers, and concomitantly reduced the expression of E-cadherin, an epithelial marker ( Fig. 1a ). Similar results were obtained in MDA-MB-468 cells in response to EGF treatment ( Fig. 1a ), suggesting that different EMT inducers enhance the expression of PYK2 in human mammary cells. 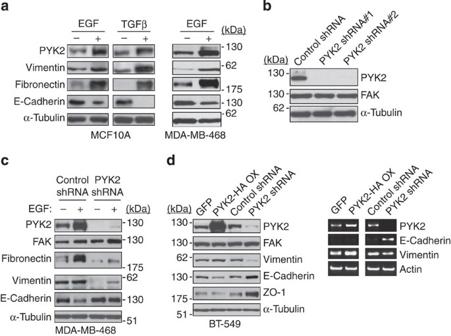Figure 1: PYK2 is upregulated during EMT and affects EMT markers expression. (a) The protein level of PYK2 is elevated during EMT. MCF10A cells were grown with either TGFβ (5 ng ml−1) or EGF (10 ng ml−1) for 5 days, whereas MDA-MB-468 cells were treated with EGF (50 ng ml−1) for 72 h to induce EMT. The protein level of PYK2 and of the indicated EMT markers was examined by WB. (b) Knockdown of PYK2 expression by shRNAs. MDA-MB-468 cells were infected with lentiviruses encoding two different shRNAs (#1 and #2) against PYK2. Knockdown efficiency and specificity was assessed by WB utilizing anti-PYK2 and anti-FAK antibodies. (c) PYK2 affects EMT in MDA-MB-468. MDA-MB-468 cells were infected with control or PYK2 shRNA (#1). The cells were treated with EGF (50 ng ml−1) for 72 h to induce EMT, lysed and assessed for the expression of PYK2 and the indicated EMT markers by WB. (d) BT-549 cells were infected with lentiviruses encoding either PYK2-HA or PYK2 shRNA. The effect of PYK2 expression on the indicated EMT markers was assessed by WB or by RT–PCR (right panel). Shown are the representative results of at least three independent experiments. The uncropped western blotting images are shown inSupplementary Fig 8. Figure 1: PYK2 is upregulated during EMT and affects EMT markers expression. ( a ) The protein level of PYK2 is elevated during EMT. MCF10A cells were grown with either TGFβ (5 ng ml −1 ) or EGF (10 ng ml −1 ) for 5 days, whereas MDA-MB-468 cells were treated with EGF (50 ng ml −1 ) for 72 h to induce EMT. The protein level of PYK2 and of the indicated EMT markers was examined by WB. ( b ) Knockdown of PYK2 expression by shRNAs. MDA-MB-468 cells were infected with lentiviruses encoding two different shRNAs (#1 and #2) against PYK2. Knockdown efficiency and specificity was assessed by WB utilizing anti-PYK2 and anti-FAK antibodies. ( c ) PYK2 affects EMT in MDA-MB-468. MDA-MB-468 cells were infected with control or PYK2 shRNA (#1). The cells were treated with EGF (50 ng ml −1 ) for 72 h to induce EMT, lysed and assessed for the expression of PYK2 and the indicated EMT markers by WB. ( d ) BT-549 cells were infected with lentiviruses encoding either PYK2-HA or PYK2 shRNA. The effect of PYK2 expression on the indicated EMT markers was assessed by WB or by RT–PCR (right panel). Shown are the representative results of at least three independent experiments. The uncropped western blotting images are shown in Supplementary Fig 8 . Full size image To examine whether PYK2 plays a role in EGF-induced EMT in MDA-MB-468 cells, we knocked down its expression by two different short hairpin RNAs (shRNAs). These two shRNAs were expressed in lentiviral vectors and efficiently reduced the expression of PYK2 without detectable effects on FAK expression ( Fig. 1b ). As shown in Fig. 1c , the depletion of PYK2 substantially reduced the effects of EGF on vimentin, fibronectin and E-cadherin expression, suggesting that PYK2 is functionally involved in EGF-induced EMT in these cells. 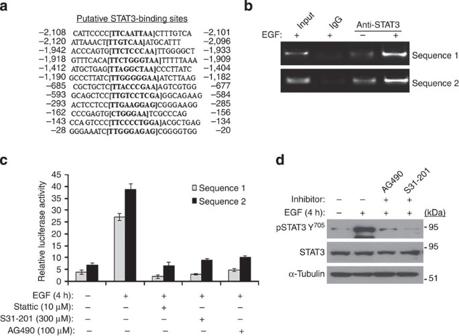Figure 8: STAT3 binds to PYK2 promoter and regulates PYK2 transcription. (a) Putative STAT3-binding sites on human PYK2 promoter are labelled in bold letters. The numbers represent the location of the indicated sequences relative to ATG. (b) ChIP analysis was performed on EGF-treated and untreated MDA-MB-468 cells using anti-STAT3 antibody and normal rabbit IgG as a negative control. Two PCR fragments were obtained in the STAT3 immunoprecipitations but not in the control IgG. The intensity of the PCR fragments was much higher in the EGF-treated samples (c) Luciferase reporter assay for PYK2 promoter activity. MDA-MB-468 cells were co-transfected with either a control pGL2-basic plasmid or with the PYK2 promoter-luciferase reporter constructs (sequence 1 or 2) together with a β-galactosidase encoding plasmid. The cells were pretreated for 1 h with dimethylsulphoxide (control) or with the indicated STAT3 inhibitors; Stattic (10 μM), S31-201 (300 μM) or AG490 (100 μM) and then stimulated with EGF for 4 h. Luciferase activity was measured by luminometer and was normalized with β-GAL activity. Fold change of luciferase activity was calculated relative to control cells transfected with the pGL2-basic plasmid. The mean values±s.d. of three independent experiments are presented in the graph. (d) S31-201 and AG490 inhibits STAT3 (Y705) phosphorylation in response to EGF. Serum-starved MDA-MB-468 cells were pretreated with S31-201 or AG490 for 1 h and then stimulated with EGF (100 ng ml−1) for 4 h. The phosphorylation of STAT3(pY705) was assessed by WB using antibodies against the indicated proteins. The uncropped western blotting images are shown inSupplementary Fig 12. To further examine the role of PYK2 in EMT, we either knocked down or overexpressed PYK2 in the mesenchymal-like human breast cancer cell line BT-549 (ref. 31 ) and assessed its influence on mesenchymal-to-epithelial transition (MET). As shown in Fig. 1d , the knockdown of PYK2 markedly enhanced the protein and/or mRNA expression of the two epithelial markers E-cadherin and ZO-1 and concomitantly reduced the expression of vimentin, while overexpression of PYK2 enhanced vimentin expression. The influence of PYK2 on the mRNA expression levels of these EMT markers was assessed by both semiquantitative reverse transcription-PCR (RT–PCR; Fig. 1d , Supplementary Fig. 1a ) and by real-time PCR (qRT–PCR, Supplementary Fig. 1b ) and similar effects were obtained. Collectively, these results suggest that PYK2 positively regulates EMT in different mammary cells. PYK2 affects breast cancer cell migration and EMT The marked effect of PYK2 depletion on the expression of E-cadherin and ZO-1 in BT-549 cells ( Fig. 1d ) led us to examine its influence on cell migration and invasion utilizing the wound healing and the matrigel invasion assays, respectively. As shown in Fig. 2a,b , the depletion of PYK2 markedly attenuated the migration and the invasion of BT-549 cells, whereas the overexpression of PYK2 enhanced cell invasion. Importantly, PYK2 depletion also reduced the expression of MMP-10 ( Supplementary Fig. 1 ) and markedly affected the characteristic elongated mesenchymal-like morphology of BT-549 cells ( Fig. 2c ). These observations are consistent with the effect of PYK2 on cell invasion ( Fig. 2b ) as well as on the expression of E-cadherin and ZO-1 that regulate cell–cell contact through adherens and tight junctions, respectively ( Fig. 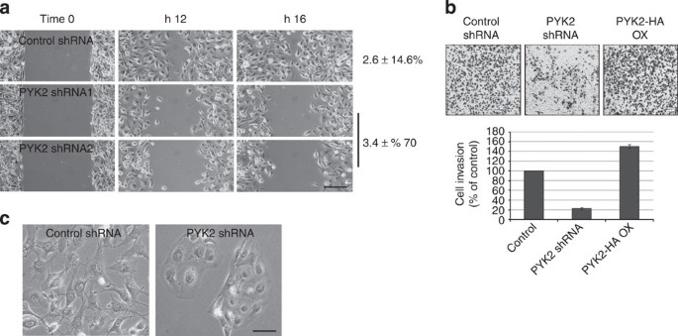1d ). Figure 2: PYK2 affects the migration, invasion and morphology of BT-549 cells. (a) PYK2 affects collective migration in BT-549 cells. Migration of control and PYK2-depleted BT-549 cells was examined by the wound-closure assay. (b) BT-549 cells were infected with lentiviruses encoding either PYK2-HA or PYK2 shRNA. The effects of PYK2 expression on cell invasion was assessed by the Matrigel-coated Boyden Chamber assay. Shown are the representative results of three independent experiments. (c) PYK2 affects BT-549 cell morphology. Bright-field micrographs of control and PYK2-depleted BT-549 cells. Scale bar, 10 μm. Figure 2: PYK2 affects the migration, invasion and morphology of BT-549 cells. ( a ) PYK2 affects collective migration in BT-549 cells. Migration of control and PYK2-depleted BT-549 cells was examined by the wound-closure assay. ( b ) BT-549 cells were infected with lentiviruses encoding either PYK2-HA or PYK2 shRNA. The effects of PYK2 expression on cell invasion was assessed by the Matrigel-coated Boyden Chamber assay. Shown are the representative results of three independent experiments. ( c ) PYK2 affects BT-549 cell morphology. Bright-field micrographs of control and PYK2-depleted BT-549 cells. Scale bar, 10 μm. Full size image We then examined whether PYK2 depletion also influences EGF-induced cell migration and invasion in MDA-MB-468 cells applying the transwell migration and invasion assays. As shown in Fig. 3a,b , the depletion of PYK2 markedly attenuated both the migration and the invasion of these cells in response to EGF. Consistent with these inhibitory effects, PYK2-depleted MDA-MB-468 cells retained their cell–cell contacts as determined by E-cadherin staining ( Fig. 3c , lower panel) and also the characteristic epithelial cell morphology even 72 h following EGF treatment ( Fig. 3c , upper panel). Overexpression of PYK2, on the other hand, caused the dissociation of E-cadherin from cell–cell contacts even in the absence of EGF and induced its redistribution into cytosolic punctate structures, possibly routing for lysosomal degradation [32] . Similar effects were obtained with β-Catenin staining ( Supplementary Fig. 2 ), which were accompanied by marked changes in β-Catenin phosphorylation on Tyr654, a known phosphorylation site for Src kinases [33] . These profound effects of PYK2 on the distribution of both E-cadherin and β-Catenin could be mediated directly by PYK2 (ref. 34 ) or possibly indirectly by Src activation. 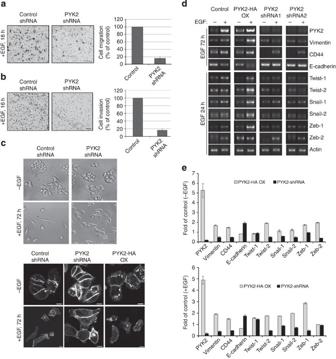It was previously shown that activated Src phosphorylates E-cadherin and/or β-Catenin, thereby facilitating the dissociation of cadherin–catenins complexes and enhancing the breakdown of adherens junctions [35] . Figure 3: PYK2 affects EGF-induced migration, invasion and EMT in MDA-MB-468 cells. (a) The influence of PYK2 depletion on EGF-induced migration of MDA-MB-468 cells was assessed by the Boyden Chamber assay as described in Methods. (b) The effect of PYK2 depletion on EGF-induced invasion of MDA-MB-468 cells through matrigel was assessed by Boyden Chamber assay. Representative images of the migrated and invaded cells are shown (a,b) along with plotted graphs demonstrating the mean values±s.d. from three independent experiments. Scale bar, 100 μm. (c) PYK2 affects EGF-induced morphological changes in MDA-MB-468 cells. Control or PYK2-depleted MDA-MB-468 cells were treated with EGF (50 ng ml−1) for 72 h to induce EMT. The phase-contrast images in the upper panels demonstrate the characteristic morphology of the cells in the absence or presence of EGF and/or PYK2 expression. The confocal images in the lower panel demonstrate the effect of PYK2 depletion or its overexpression on cell–cell contact using E-cadherin staining. Scale bar, 10 μm. (d,e) The mRNA expression levels of PYK2 and the indicated EMT markers as well as transcription factors were examined by semiquantitative RT–PCR (d) and by real-time PCR (qRT–PCR). (e) Shown are the representative results of three independent experiments demonstrating the effect of EGF in control and in PYK2-depleted or overexpressed MDA-MB-468 cells. The intensity of the RT–PCR bands was assessed by densitometry (Image J) and mean values±s.d. were calculated and are presented inSupplementary Table 2. The mean values of the qRT–PCR±s.d. were calculated (Supplementary Table 3) and are presented as fold of control values. Figure 3: PYK2 affects EGF-induced migration, invasion and EMT in MDA-MB-468 cells. ( a ) The influence of PYK2 depletion on EGF-induced migration of MDA-MB-468 cells was assessed by the Boyden Chamber assay as described in Methods. ( b ) The effect of PYK2 depletion on EGF-induced invasion of MDA-MB-468 cells through matrigel was assessed by Boyden Chamber assay. Representative images of the migrated and invaded cells are shown ( a , b ) along with plotted graphs demonstrating the mean values±s.d. from three independent experiments. Scale bar, 100 μm. ( c ) PYK2 affects EGF-induced morphological changes in MDA-MB-468 cells. Control or PYK2-depleted MDA-MB-468 cells were treated with EGF (50 ng ml −1 ) for 72 h to induce EMT. The phase-contrast images in the upper panels demonstrate the characteristic morphology of the cells in the absence or presence of EGF and/or PYK2 expression. The confocal images in the lower panel demonstrate the effect of PYK2 depletion or its overexpression on cell–cell contact using E-cadherin staining. Scale bar, 10 μm. ( d , e ) The mRNA expression levels of PYK2 and the indicated EMT markers as well as transcription factors were examined by semiquantitative RT–PCR ( d ) and by real-time PCR (qRT–PCR). ( e ) Shown are the representative results of three independent experiments demonstrating the effect of EGF in control and in PYK2-depleted or overexpressed MDA-MB-468 cells. The intensity of the RT–PCR bands was assessed by densitometry (Image J) and mean values±s.d. were calculated and are presented in Supplementary Table 2 . The mean values of the qRT–PCR±s.d. were calculated ( Supplementary Table 3 ) and are presented as fold of control values. Full size image Loss of E-cadherin is thought to be the prototypical marker of EMT [36] and is known to be regulated at both the transcriptional and post-transcriptional levels [37] . Several transcriptional factors, including Snail, Slug, Zeb-1 (ref. 38 ) and Twist [39] , repress the expression of E-cadherin. These transcription factors play central roles in EMT during embryogenesis and are implicated in cancer progression [40] . We therefore examined the influence of PYK2 on the mRNA levels of these transcription factors using RT–PCR ( Fig. 3d and Supplementary Table 2 ) and qRT–PCR ( Fig. 3e and Supplementary Table 3 ). As shown, the overexpression of PYK2 in MDA-MB-468 cells significantly enhanced the inducible effect of EGF on Twist-2, Snail-1,2 and Zeb-1,2 expression, whereas the knockdown of PYK2 had opposite effects. These results were consistent with the influence of PYK2 on the mRNA level of E-cadherin as well as on the levels of vimentin and CD44 ( Fig. 3d,e and Supplementary Tables 2,3 ). In BT-549 cells, PYK2 had less profound effects on these transcription factors. Yet, its overexpression enhanced the expression of Snail2 and Zeb-2 ( Supplementary Fig. 1 ). Altogether, our results suggest that PYK2 expression enhances EMT at both the cellular and the molecular levels. PYK2 expression correlates with tumour grade and metastasis Elevated expression of several EMT transcription factors has been considered as biomarker for lymph node metastasis (LNM) and poor prognosis in many human cancers including breast cancer [41] , [42] . The marked influence of PYK2 on the expression level of EMT transcription factors in MDA-MB-468 and BT-549 cells ( Fig. 3d,e , Supplementary Fig. 1 and Supplementary Tables 2,3 ) led us to examine its expression in normal breast tissue and breast cancer samples of patients with different tumour grade and LNM status. The expression of PYK2 was determined by immunohistochemistry (IH) analysis of 92 paraffin-embedded sections of human breast cancer samples. The results revealed a significantly higher number (79.3%, 73/92) of cancer samples with high-to-moderate PYK2 staining. No staining or very weak staining of PYK2 was observed in adjacent non-tumour tissue and all normal samples ( Fig. 4 ). Most importantly, we found that 76% (41/54) of high-grade tumours show high PYK2 staining ( P =0.019, χ 2 -statistics, Fig. 4b ), and that PYK2 expression is significantly correlated with LNM status. Of the total 92 breast cancer samples, 28 samples were lymph node positive, of which 26 (92.8%) had high-to-moderate PYK2 expression ( P =0.034). These results suggest that PYK2 expression correlates with both high-grade tumours and early metastatic events. 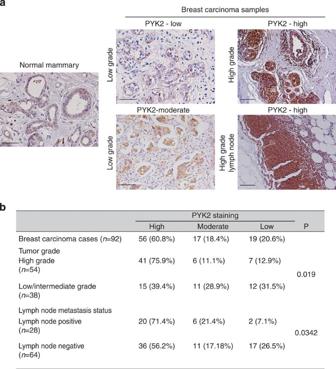Collectively, these results suggest that PYK2 not only affects cell migration, invasion and EMT in cellular models in vitro , but most likely enhances breast cancer progression and metastasis in human patients. Figure 4: High expression of PYK2 is associated with high histological tumour grade and LNM. (a) Immunohistochemical analysis of PYK2 expression in normal mammary tissue and breast cancer samples of different tumour grades and lymph node status. Representative pictures are shown. Staining intensity of PYK2 was classified as high, moderate or low as described in Methods. Scale bar, 50 μm. (b) Quantitative evaluation of 92 breast cancer patient samples for PYK2 expression was performed using H-score (H-Score=ΣPi, (i+1), wherePiis the percentage of stained cells in each intensity category andiis the relative intensity;i=1, 2, 3). The correlations between PYK2 expression and tumor grade or LNM status are shown. Statistical analysis was performed byχ2-analysis. Figure 4: High expression of PYK2 is associated with high histological tumour grade and LNM. ( a ) Immunohistochemical analysis of PYK2 expression in normal mammary tissue and breast cancer samples of different tumour grades and lymph node status. Representative pictures are shown. Staining intensity of PYK2 was classified as high, moderate or low as described in Methods. Scale bar, 50 μm. ( b ) Quantitative evaluation of 92 breast cancer patient samples for PYK2 expression was performed using H-score (H-Score=Σ P i , ( i +1), where P i is the percentage of stained cells in each intensity category and i is the relative intensity; i =1, 2, 3). The correlations between PYK2 expression and tumor grade or LNM status are shown. Statistical analysis was performed by χ 2 -analysis. Full size image PYK2 modulates EGF-induced EMT signalling Thus far, we show that PYK2 expression correlates with high-grade breast tumours and enhances EMT in vitro . To gain mechanistic insight into the role of PYK2 in EMT, we examined its influence on EGF-induced signalling in MDA-MB-468 cells. Application of EGF to these cells induced rapid tyrosine phosphorylation of PYK2 (within 3 min; Fig. 5a ), which was sustained for more than 20 h. This rapid phosphorylation was associated with a redistribution of phospho-PYK2 (pY402) from peripheral focal adhesions into punctate cytosolic structures, observed 30–60 min following EGF treatment ( Fig. 5b ). Importantly, these cytosolic structures failed to co-localize with the focal adhesion protein paxillin but extensively co-localized with EGFR ( Fig. 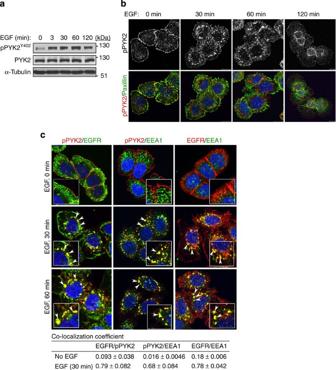5b,c ). Figure 5: EGF induces PYK2 phosphorylation, translocation of PYK2 to early endosomes and its co-localization with EGFR. (a) MDA-MB-468 cells were serum starved for 24 h and then stimulated with EGF (100 ng ml−1) for the indicated time periods. Total cell lysates were analysed for PYK2 phosphorylation on Y402 by WB analysis using the anti-pPYK2 (Y402) antibody. (b) Subcellular localization of pPYK2 (Y402). Serum-starved MDA-MB-468 cells were stimulated with EGF (100 ng ml−1) for the indicated time points. The cells were then fixed and double immunostained with anti-pPYK2 (Y402) (red) and anti-paxillin (green) antibodies. Shown are representative confocal images. Scale bar, 10 μm. (c) EGFR and pPYK2 (Y402) co-localize on early endosomes. The localization of EGFR, pPYK2 (Y402) and the early endosomal marker EEA1 was examined by immunofluorescence analysis. Shown are the representative confocal images. Co-localization appears in yellow. Scale bar, 10 μm. Co-localization was measured as described in ‘Methods’ and Manders’ co-localization coefficient was calculated. Shown are the mean values of the co-localization coefficient±s.d. from >20 cells. The uncropped western blotting images are shown inSupplementary Fig 9. Figure 5: EGF induces PYK2 phosphorylation, translocation of PYK2 to early endosomes and its co-localization with EGFR. ( a ) MDA-MB-468 cells were serum starved for 24 h and then stimulated with EGF (100 ng ml −1 ) for the indicated time periods. Total cell lysates were analysed for PYK2 phosphorylation on Y402 by WB analysis using the anti-pPYK2 (Y402) antibody. ( b ) Subcellular localization of pPYK2 (Y402). Serum-starved MDA-MB-468 cells were stimulated with EGF (100 ng ml −1 ) for the indicated time points. The cells were then fixed and double immunostained with anti-pPYK2 (Y402) (red) and anti-paxillin (green) antibodies. Shown are representative confocal images. Scale bar, 10 μm. ( c ) EGFR and pPYK2 (Y402) co-localize on early endosomes. The localization of EGFR, pPYK2 (Y402) and the early endosomal marker EEA1 was examined by immunofluorescence analysis. Shown are the representative confocal images. Co-localization appears in yellow. Scale bar, 10 μm. Co-localization was measured as described in ‘Methods’ and Manders’ co-localization coefficient was calculated. Shown are the mean values of the co-localization coefficient±s.d. from >20 cells. The uncropped western blotting images are shown in Supplementary Fig 9 . Full size image Numerous studies described the critical role of RTK endocytosis for downstream signalling and cellular responses. 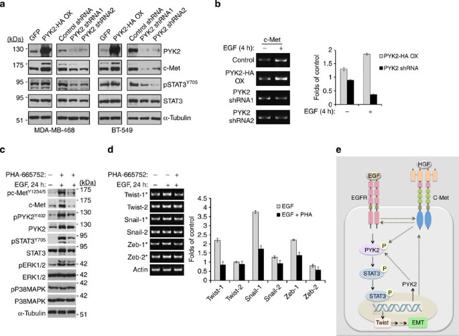Figure 9: Positive feedback in the PYK2–STAT3–c-MET axis. (a) PYK2 depletion or its overexpression affects the steady-state level of c-Met protein as well as the phosphorylation of STAT3 in MDA-MB-468 and BT-549 cells as determined by WB analysis. (b) PYK2 affects EGF-induced upregulation of c-Met mRNA in MDA-MB-468 cells as determined by RT–PCR (left panel) and by real-time PCR (qRT–PCR; graph, right panel). Overexpression (OX). (c) The c-Met inhibitor PHA-66752 (10 μM) reduces the phosphorylation of STAT3 and PYK2 in response to EGF (24 h) and also of the mRNA levels of EMT transcription factors as determined by WB analysis (c) and by RT–PCR (d, left panel) or qRT–PCR (d, graph), respectively. The intensity of the RT–PCR bands was assessed by densitometry (Image J). Mean values of qRT–PCR±s.d. were calculated and presented in the graph as fold of control EGF-untreated values. (e) A scheme depicting the positive feedback loop between EGFR/c-Met, PYK2 and STAT3. EGFR and c-Met, which cantrans-phosphorylate each other, activate PYK2 (PY402), which in turn, enhances STAT3 phosphorylation (pY705). Phospho-STAT3(pY705) translocates to the nucleus, binds to PYK2 prompter and enhances its transcription. pSTAT3 also enhances the expression of c-Met, possibly indirectly, and of Twist, which is required for EMT. The uncropped western blotting images are shown inSupplementary Fig 13. The canonical model involves rapid internalization of a ligand-activated RTK at the cell surface by clathrin-dependent or -independent endocytosis, fusion with early endosomes and sorting of the internalized receptor to lysosomes for degradation and signalling termination [6] . To define the cytosolic structures at which phospho-PYK2 (pY402) and EGFR were co-localized, we co-stained EGF-treated MDA-MB-468 cells with the early endosomal marker EEA1 or the lysosomal marker LAMP3 together with either EGFR or pPYK2 (pY402). As seen in Fig. 5c , both EGFR and pPYK2 (pY402) were detected at early endosomes 30–60 min after EGF treatment. Their co-localization with EEA1 was measured as described in Methods and found to be significantly high ( P <0.001, Fig. 5c ). No detectable co-localization with LAMP3 was obtained. These results suggest that activated PYK2 co-localizes with RTKs on early endosomes. We then asked whether PYK2 affects EGF-mediated signalling pathways. As shown in Fig. 6a , EGF induces the rapid activation (within 3 min) of multiple signalling pathways including the MAPK (mitogen-activated protein kinase) pathway, PI3K/AKT pathway as well as the signal transducer and activator of transcription 3 (STAT3) pathway. Depletion of PYK2 substantially inhibited STAT3 and ERK1/2 phosphorylation, but had no obvious effect on AKT phosphorylation. To examine whether PYK2 exerts transient effect on STAT3 and ERK1/2 phosphorylation, we assessed their phosphorylation in response to EGF treatment for up to 2 h. As shown in Fig. 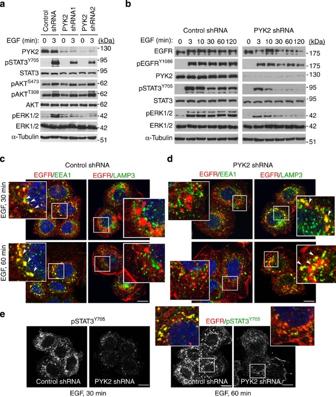6b , the depletion of PYK2 substantially reduced the phosphorylation of STAT3 and ERK1/2 over time, and most importantly, reduced the protein level of EGFR 30–120 min following EGF treatment. These results suggest that depletion of PYK2 facilitates the degradation of the receptor. Figure 6: Depletion of PYK2 inhibits EGFR downstream signalling and accelerates EGFR lysosomal targeting. (a,b) PYK2 depletion affects EGFR downstream signalling. Control and PYK2-depleted MDA-MB-468 cells were serum starved for 24 h and then stimulated with EGF (100 ng ml−1) for the indicated time points. The activation of different signalling pathways downstream of EGFR was assessed by WB using the indicated antibodies. The protein level of EGFR was assessed by WB using anti-EGFR antibody (b). (c,d) PYK2 depletion accelerates the lysosomal targeting of EGFR. The localization of EGFR on early endosomes or lysosomes in control (c) or PYK2-depleted cells (d) was determined by co-staining with anti-EGFR antibody and either anti-EEA1 or anti-Lamp3 antibodies, respectively. Shown are the representative confocal images. Co-localization appears in yellow. Scale bar, 10 μm. (e) Phospho-STAT3Y705co-localizes with EGFR on endosomal-like structures 30–60 min following EGF treatment of control, but not of PYK2-depleted MDA-MB-468 cells. Scale bar, 10 μm. The uncropped western blotting images are shown inSupplementary Fig 10. Figure 6: Depletion of PYK2 inhibits EGFR downstream signalling and accelerates EGFR lysosomal targeting. ( a , b ) PYK2 depletion affects EGFR downstream signalling. Control and PYK2-depleted MDA-MB-468 cells were serum starved for 24 h and then stimulated with EGF (100 ng ml −1 ) for the indicated time points. The activation of different signalling pathways downstream of EGFR was assessed by WB using the indicated antibodies. The protein level of EGFR was assessed by WB using anti-EGFR antibody ( b ). ( c , d ) PYK2 depletion accelerates the lysosomal targeting of EGFR. The localization of EGFR on early endosomes or lysosomes in control ( c ) or PYK2-depleted cells ( d ) was determined by co-staining with anti-EGFR antibody and either anti-EEA1 or anti-Lamp3 antibodies, respectively. Shown are the representative confocal images. Co-localization appears in yellow. Scale bar, 10 μm. ( e ) Phospho-STAT3 Y705 co-localizes with EGFR on endosomal-like structures 30–60 min following EGF treatment of control, but not of PYK2-depleted MDA-MB-468 cells. Scale bar, 10 μm. The uncropped western blotting images are shown in Supplementary Fig 10 . Full size image To explore this possibility, we first examined the subcellular localization of EGFR in the control and PYK2-depleted MDA-MB-468 cells 30–60 min following EGF treatment. As shown, EGFR clearly localized to early endosomes (EEA1 positive) in control cells ( Fig. 6c ), but extensively co-localized with the lysosomal marker LAMP3 in PYK2-depleted cells ( Fig. 6d ; co-localization coefficient of EGFR/LAMP3 was 0.75±0.1, P <0.001). Strikingly, at this time point, no detectable co-localization of EGFR and LAMP3 was observed in the control cells, suggesting that the depletion of PYK2 facilitates the lysosomal targeting of the receptor and its subsequent degradation. Consistent with this possibility, the knockdown of PYK2 enhanced receptor ubiquitination in response to EGF treatment ( Supplementary Fig. 3 ). Moreover, immunofluorescence analysis of EGFR and its downstream effector phospho-STAT3 (pY705) clearly demonstrated their co-localization at endosomal-like structures in control MDA-MB-468 cells 30–60 min following EGF treatment (co-localization coefficient of EGFR/pSTAT3 was 0.748±0.043, P <0.001). This co-localization was not observed in PYK2-depleted cells ( Fig. 6e ), suggesting that PYK2 not only localizes at early endosomes on EGF stimulation, but also influences endosomal-derived receptor signalling. Indeed, we could detect association between PYK2, EGFR and STAT3 in response to EGF treatment using co-immunoprecipitation studies ( Supplementary Fig. 4 ). These results suggest that these three proteins interact directly or indirectly with one another at the endosomal compartment, and that activated PYK2 links EGFR to its downstream effectors and sustains endosomal-derived receptor signalling. STAT3 phosphorylation is essential for EGF-induced EMT The marked effect of PYK2 on STAT3 phosphorylation (pY705; Fig. 6a,b ) together with its influence on EMT ( Fig. 1c ) suggests that STAT3 phosphorylation is essential for EGF-induced EMT in MDA-MB-468 cells. To examine this possibility, we inhibited STAT3 phosphorylation using the JAK2/STAT3 inhibitor AG490. This inhibitor abolished the phosphorylation of STAT3 (pY705) in response to EGF treatment ( Fig. 7c ) and concomitantly reduced the positive or negative effects of EGF on mesenchymal (CD44, vimentin and fibronectin) or epithelial (E-cadherin, ZO-1) markers, respectively ( Fig. 7a ). Consistent with these effects on EMT markers, AG490 almost completely abolished the typical morphological changes of EGF-treated MDA-MB-468 cells, and instead the cells maintained their characteristic epithelial shape ( Fig. 7b ). 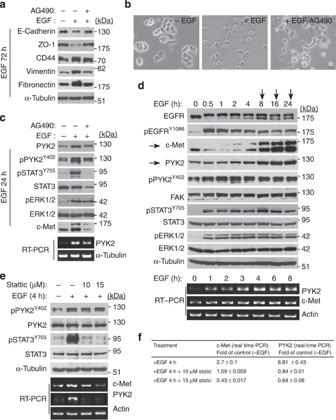Furthermore, AG490 also decreased the inducible effects of EGF on the protein, mRNA and phosphorylation (pY402) levels of PYK2 ( Fig. 7c ). Figure 7: STAT3 activation is required for EGF-induced EMT and for the upregulation of PYK2 and c-Met expression. (a) The JAK/STAT3 inhibitor AG490 reduces the effects of EGF on EMT markers in MDA-MB-468 cells. Serum-starved MDA-MB-468 cells were pretreated with AG490 (50 μM) for 1 h and then stimulated with EGF (50 ng ml−1) for the indicated time periods. The level of the indicated EMT marker proteins was assessed by WB using the corresponding antibodies. (b) AG490 prevents EGF-induced morphological changes in MDA-MB-468 cells. Shown are the representative bright-field micrographs of control and EGF-treated cells for 24 h in the absence or presence of AG490. Scale bar, 10 μm. (c) AG490 reduced the effects of EGF on STAT3 phosphorylation, on the protein level of PYK2 and c-Met, and on the mRNA level PYK2 as determined by WB and RT–PCR analysis, respectively. (d) PYK2 and c-Met are concurrently upregulated in EGF-treated MDA-MB-468 cells. The protein levels of c-Met and PYK2 as well as the indicated signalling proteins were assessed by WB (upper panel) at different time points following EGF stimulation. The mRNA levels of c-Met and PYK2 was examined by RT–PCR (lower panels). (e,f) The STAT3 inhibitor Stattic (10–15 μM) abolished or reduced the effect of EGF (4 h) on PYK2 or c-Met mRNA expression, respectively, as determined by RT–PCR (e) and by real-time PCR (f). Reproducible results were obtained in three independent experiments and mean values of qRT–PCR±s.d were calculated. Results are presented as fold of control. The uncropped western blotting images are shown inSupplementary Fig 11. Figure 7: STAT3 activation is required for EGF-induced EMT and for the upregulation of PYK2 and c-Met expression. ( a ) The JAK/STAT3 inhibitor AG490 reduces the effects of EGF on EMT markers in MDA-MB-468 cells. Serum-starved MDA-MB-468 cells were pretreated with AG490 (50 μM) for 1 h and then stimulated with EGF (50 ng ml −1 ) for the indicated time periods. The level of the indicated EMT marker proteins was assessed by WB using the corresponding antibodies. ( b ) AG490 prevents EGF-induced morphological changes in MDA-MB-468 cells. Shown are the representative bright-field micrographs of control and EGF-treated cells for 24 h in the absence or presence of AG490. Scale bar, 10 μm. ( c ) AG490 reduced the effects of EGF on STAT3 phosphorylation, on the protein level of PYK2 and c-Met, and on the mRNA level PYK2 as determined by WB and RT–PCR analysis, respectively. ( d ) PYK2 and c-Met are concurrently upregulated in EGF-treated MDA-MB-468 cells. The protein levels of c-Met and PYK2 as well as the indicated signalling proteins were assessed by WB (upper panel) at different time points following EGF stimulation. The mRNA levels of c-Met and PYK2 was examined by RT–PCR (lower panels). ( e , f ) The STAT3 inhibitor Stattic (10–15 μM) abolished or reduced the effect of EGF (4 h) on PYK2 or c-Met mRNA expression, respectively, as determined by RT–PCR ( e ) and by real-time PCR ( f ). Reproducible results were obtained in three independent experiments and mean values of qRT–PCR±s.d were calculated. Results are presented as fold of control. The uncropped western blotting images are shown in Supplementary Fig 11 . Full size image In many cancer cells, the EGF also induces the expression of the HGF receptor c-Met [43] . Both EGFR and c-Met are involved in EMT and implicated in the tumorigenesis and metastasis of different human cancers including glioblastoma, small lung carcinoma and breast cancer [44] , [45] . Strikingly, we found that EGF caused an upregulation of c-Met expression and that AG490 abolished this effect ( Fig. 7c ), suggesting that STAT3 phosphorylation not only affects the expression of PYK2 but also influences c-Met expression. To better characterize the effect of EGF on PYK2 and c-Met expression, we examined their protein and mRNA levels in MDA-MB-468 cells at different time points following EGF stimulation using western blotting (WB) and RT–PCR, respectively. As shown in Fig. 7d , a substantial upregulation of PYK2 and c-Met protein expression was detected ~8 h following EGF stimulation. Notably, we did not detect corresponding upregulation in FAK protein for up to 24 h, suggesting that PYK2 and FAK are distinctly regulated in these cells. RT–PCR analysis revealed a remarkable upregulation of PYK2 mRNA within 1 h following EGF treatment, which was further increased to maximal level at 4 h. Peak of c-Met mRNA expression level was also observed at 4 h following EGF treatment ( Fig. 7d , lower panel). To examine whether STAT3 phosphorylation is also required for EGF-induced PYK2 and c-Met mRNA expression, we used the STAT3-specific inhibitor Stattic [46] , [47] . As seen, Stattic completely abolished both the phosphorylation of STAT3 (pY705; Fig. 7e ) and the upregulation of PYK2 transcription in response to EGF as determined by RT–PCR ( Fig. 7e ) and by qRT–PCR ( Fig. 7f ). However, it partially inhibited the EGF-induced c-Met expression ( Fig. 7e,f ). It is worth mentioning that Stattic has toxic effects over time (longer than 12 h) and therefore its effects on EMT markers could not been assessed. STAT3 directly regulates PYK2 transcription The profound effect of Stattic on PYK2 mRNA level ( Fig. 7e,f ) raised the possibility that STAT3 directly regulates PYK2 transcription. To examine this possibility, we searched for canonical STAT3-binding motifs TTC(N) 2–4 GAA or TT(N) 4–6 AA (refs 48 , 49 ) within the promoter region of PYK2. Several putative sites have been identified ( Fig. 8a ) and PCR primers were designed accordingly ( Supplementary Table 4 ). To examine whether these sites bind STAT3 in vivo , we applied chromatin immunoprecipitation (ChIP) of control and EGF-treated MDA-MB-468 cells. Two of the four PCR fragments containing the putative STAT3-binding motifs were obtained in the anti-STAT3 immunoprecipitation but not in the control normal immunoglobulin G (IgG). Moreover, much stronger amplification of the PCR fragments was observed in the EGF-induced samples ( Fig. 8b ), consistent with the upregulation of PYK2 transcription in response to EGF treatment ( Fig. 7c–e ). Sequence analysis confirmed that these two fragments were amplified from PYK2 promoter. Subsequently, the two PCR fragments were subcloned upstream of the luciferase reporter gene and expressed in MDA-MB-468 cells. The cells were then stimulated with EGF in the absence or presence of three different STAT3 inhibitors Stattic (10 μM), S31-201 (300 μM) and AG490 (100 μM) (refs 47 , 50 ), which effectively inhibit STAT3 phosphorylation (pY 705 ; Figs 7e and 8d ). As seen in Fig. 8c , high luciferase activity was detected with both fragments in response to EGF treatment, which was almost abolished in the presence of the STAT3 inhibitors. These results are consistent with the ChIP analysis and strongly suggest that STAT3 directly regulates the transcription of PYK2 via these two binding sites at the proximal promoter region of the human PYK2 gene. Figure 8: STAT3 binds to PYK2 promoter and regulates PYK2 transcription. ( a ) Putative STAT3-binding sites on human PYK2 promoter are labelled in bold letters. The numbers represent the location of the indicated sequences relative to ATG. ( b ) ChIP analysis was performed on EGF-treated and untreated MDA-MB-468 cells using anti-STAT3 antibody and normal rabbit IgG as a negative control. Two PCR fragments were obtained in the STAT3 immunoprecipitations but not in the control IgG. The intensity of the PCR fragments was much higher in the EGF-treated samples ( c ) Luciferase reporter assay for PYK2 promoter activity. MDA-MB-468 cells were co-transfected with either a control pGL2-basic plasmid or with the PYK2 promoter-luciferase reporter constructs (sequence 1 or 2) together with a β-galactosidase encoding plasmid. The cells were pretreated for 1 h with dimethylsulphoxide (control) or with the indicated STAT3 inhibitors; Stattic (10 μM), S31-201 (300 μM) or AG490 (100 μM) and then stimulated with EGF for 4 h. Luciferase activity was measured by luminometer and was normalized with β-GAL activity. Fold change of luciferase activity was calculated relative to control cells transfected with the pGL2-basic plasmid. The mean values±s.d. of three independent experiments are presented in the graph. ( d ) S31-201 and AG490 inhibits STAT3 (Y 705 ) phosphorylation in response to EGF. Serum-starved MDA-MB-468 cells were pretreated with S31-201 or AG490 for 1 h and then stimulated with EGF (100 ng ml −1 ) for 4 h. The phosphorylation of STAT3(pY 705 ) was assessed by WB using antibodies against the indicated proteins. The uncropped western blotting images are shown in Supplementary Fig 12 . Full size image Positive feedback between PYK2-STAT3-c-Met Thus far, we showed that PYK2 positively regulates STAT3 phosphorylation ( Fig. 6a,b and Supplementary Fig. 5a ), which in turn, directly or indirectly, enhances the expression of PYK2 and c-Met ( Figs 7c,e and 8b , Supplementary Fig. 5b ). We also showed that both PYK2 and phospho-STAT3 positively regulate EMT in several mammary carcinoma cell lines ( Figs 1c,d , 3d and 7a,b ). Importantly, c-Met is also associated with EMT signature in triple-negative breast cancer [51] , [52] and plays a central role in breast cancer progression and metastasis [53] . Furthermore, previous studies suggest that the activation of STAT3 downstream of c-Met is crucial for cell invasion [54] , transformation and tumorigenesis [55] . These observations suggest that PYK2, STAT3 and c-Met are interdependently regulated, possibly at both the transcriptional and post-transcriptional (phosphorylation, protein degradation) levels, and positively regulate EMT in several mammary cell lines. To explore this possibility, we examined the influence of each protein of the PYK2–STAT3–c-Met axis on the other two. Since we already assessed the influence of STAT3 on c-Met and PYK2 ( Fig. 7c,e and Supplementary Fig. 5b ), and of PYK2 on STAT3 ( Fig. 6a,b,e and Supplementary Fig. 5a ), we examined the effect of PYK2 on the protein level of c-Met in MDA-MB-468 and BT-549 cells under steady-state conditions. As shown in Fig. 9a , the overexpression of PYK2 markedly increased the level of c-Met in both cell lines, while the depletion of PYK2 decreased c-Met level. We further assessed the influence of PYK2 on c-Met mRNA expression utilizing RT–PCR and qRT–PCR. Although we could not detect the obvious effect of PYK2 on the mRNA level of c-Met under steady-state conditions, its overexpression in MDA-MB-468 cells markedly enhanced the stimulatory effect of EGF on c-Met transcription, whereas PYK2 depletion had an opposite effect ( Fig. 9b ). These results suggest that in these cells PYK2 positively regulates c-Met level both at the protein and the mRNA levels. Figure 9: Positive feedback in the PYK2–STAT3–c-MET axis. ( a ) PYK2 depletion or its overexpression affects the steady-state level of c-Met protein as well as the phosphorylation of STAT3 in MDA-MB-468 and BT-549 cells as determined by WB analysis. ( b ) PYK2 affects EGF-induced upregulation of c-Met mRNA in MDA-MB-468 cells as determined by RT–PCR (left panel) and by real-time PCR (qRT–PCR; graph, right panel). Overexpression (OX). ( c ) The c-Met inhibitor PHA-66752 (10 μM) reduces the phosphorylation of STAT3 and PYK2 in response to EGF (24 h) and also of the mRNA levels of EMT transcription factors as determined by WB analysis ( c ) and by RT–PCR ( d , left panel) or qRT–PCR ( d , graph), respectively. The intensity of the RT–PCR bands was assessed by densitometry (Image J). Mean values of qRT–PCR±s.d. were calculated and presented in the graph as fold of control EGF-untreated values. ( e ) A scheme depicting the positive feedback loop between EGFR/c-Met, PYK2 and STAT3. EGFR and c-Met, which can trans -phosphorylate each other, activate PYK2 (PY402), which in turn, enhances STAT3 phosphorylation (pY705). Phospho-STAT3(pY705) translocates to the nucleus, binds to PYK2 prompter and enhances its transcription. pSTAT3 also enhances the expression of c-Met, possibly indirectly, and of Twist, which is required for EMT. The uncropped western blotting images are shown in Supplementary Fig 13 . Full size image We then asked whether c-Met affects EGF-induced PYK2 and STAT3 phosphorylation in MDA-MB-468 cells, and whether it concomitantly influences the expression of EMT transcription factors. To address these questions, we used the c-Met inhibitor PHA-665752. As seen in Fig. 9c , PHA-665752 partially inhibited the phosphorylation of PYK2 and STAT3, concurrent with its partial inhibition of EGF-induced expression of the EMT transcription factors Zeb-1/2, Twist1 and Snail-1 ( Fig. 9d ). Interestingly, the PHA-665752 inhibitor abolished the upregulation of c-Met in response to EGF, possibly by influencing PYK2 and STAT3 phosphorylation. Taken together, our results suggest that a positive feedback within the PYK2–STAT3–c-Met axis enhances EMT in mammary cells ( Fig. 9e ). In this study, we show that the non-receptor tyrosine kinase PYK2 functionally contributes to EMT in human mammary cancer cells ( Figs 1 , 2 , 3 ). We found that the expression level of PYK2 is markedly increased in response to EMT inducers ( Fig. 1a ) and that the downregulation of PYK2 inhibits EMT or enhances MET, while the overexpression of PYK2 had opposite effects ( Figs 2 and 3 ). Consistent with these findings, previous studies suggest that PYK2 induces EMT in hepatocellular carcinoma thereby promoting cell motility [23] , and that PYK2 expression is robustly upregulated during EMT in breast cancer cells [28] . However, the underlying mechanisms of these findings and their clinical implications have not been thoroughly explored. Our IH analysis of 92 clinical samples derived from 92 human breast cancer patients is possibly the most striking evidence that PYK2 expression correlates with high tumour grade and LNM ( Fig. 4 ). It is well known that LNM is mediated by EMT-associated processes, including cell migration and invasion, and is directly associated with poor prognosis [56] . Hence, our findings suggest that PYK2 not only affects EMT in cultured cells and breast cancer in animal models [28] , but also contributes to human breast cancer progression and metastasis. Mechanistically, our studies suggest that PYK2 prolongs EMT-associated signals and consequently enhances EMT. We suggest that PYK2 prolongs the signal duration by (i) sustaining endosomal-derived receptor signalling and by (ii) persisting the activation of a transcription factor through a positive feedback loop ( Fig. 9e ). In MDA-MB-468 cells, which undergo EMT in response to EGF, PYK2 co-localizes with EGFR at early endosomes shortly (30 min) after EGF treatment ( Fig. 5c ) and EGFR co-localizes with pSTAT3 ( Fig. 6e ). These results suggest that EGFR, PYK2 and pSTAT3 are localized at the same subcellular compartment in response to EGF treatment and might interact with one another. Indeed, co-immunoprecipitation studies suggest that PYK2, EGFR and pSTAT3 can be found in the same immunocomplex ( Supplementary Fig. 4 ), and, thus, directly or indirectly interact. We further found that the depletion of PYK2 facilitated the lysosomal targeting of EGFR and enhanced receptor degradation ( Fig. 6b,d and Supplementary Fig. 3 ). Interestingly, the inhibition of Src activity in these cells markedly affects receptor internalization and not receptor degradation ( Supplementary Fig. 7 ). These results are in agreement with previous reports [57] and suggest that Src acts upstream of PYK2, and that Src and PYK2 may function sequentially and regulate receptor internalization and its subsequent endosomal signalling, respectively. Indeed, PYK2 depletion markedly reduced the phosphorylation of STAT3 and ERK1/2 ( Fig. 6a,b ), which have been implicated in endosomal-derived signalling of many RTKs [58] , but had no obvious effect on AKT phosphorylation ( Fig. 6a ), which is considered to take place at the cell surface [5] . It is unclear, yet, how PYK2 sustains endosomal signalling of EGFR, and several potential mechanisms can be postulated, including interfering with the ubiquitination machinery through physical interaction with the receptor or, alternatively, through a direct influence on components of the ubiquitination machinery, such as c-Cbl, as previously described for Src [59] . Physical interfering with the ubiquitination machinery is supported by the co-localization ( Fig. 5c ) and co-immunoprecipitation ( Supplementary Fig. 4 ) studies as well as by the enhanced ubiquitination of the receptor in PYK2-depleted cells ( Supplementary Fig. 3 ), but should be further explored. Regardless of the precise mechanism, we also observed co-localization between PYK2 and c-Met at early endosomes ( Supplementary Fig. 6b ). This suggests that PYK2 plays a general role in endosomal-derived signalling of certain RTKs in specific cells. Co-localization between phospho-PYK2 (pY402) and EGFR at early endosomes was also detected in BT-20 cells in response to EGF treatment ( Supplementary Fig. 6a ). Most strikingly, EGF also induced the phosphorylation of PYK2 and c-Met and their co-localization at endosomal-like structures in MDA-MB-468 and BT-20 cells ( Supplementary Fig. 6b,d ). These results are consistent with previous studies describing the crosstalk between EGFR and c-Met, and the ability of EGFR to trans-activate c-Met [58] . In some cancers, such as non-small-cell lung cancer, the activation of EGFR not only enhances the phosphorylation of c-Met, but also increases its protein and mRNA expression levels [43] . Likewise, we also found that EGF enhances the expression of c-Met in MDA-MB-468 cells, concomitant with the upregulation in PYK2 expression ( Fig. 7d ). The upregulation of PYK2 expression appears to be directly regulated by STAT3 phosphorylation ( Fig. 7c,e ), whereas PYK2, either directly or indirectly, potentiates STAT3 phosphorylation ( Fig. 6a,b ). The crucial role of STAT3 phosphorylation for EGF-induced EMT in MDA-MB-468 cells has been attributed to its direct effect on Twist expression ( Fig. 9e ). STAT3 directly binds to the promoter region of Twist and regulates its transcription during EMT [60] . Similarly, we found that the proximal region of PYK2 promoter contains STAT3-binding sites and demonstrated that STAT3 directly regulates the transcription of PYK2 in response to EGF ( Fig. 8 ). In contrast to the direct and profound effect of STAT3 on PYK2 transcription, STAT3 only partially influenced c-Met expression ( Fig. 7e,f ). Since c-Met can be transcriptionally regulated by several different transcription factors, as well as by different microRNAs [61] , it could be that STAT3 indirectly influences c-Met transcription by modulating the expression of these regulators. Nevertheless, our studies suggest that STAT3 affects the expression of PYK2 ( Fig. 7c,e,f ) and partially of c-Met ( Fig. 7e,f ), and that PYK2 affects STAT3 phosphorylation ( Fig. 6a,b ) and also the protein ( Fig. 9a ) and mRNA ( Fig. 9b ) levels of c-Met. We postulate that PYK2 influences c-Met transcription through STAT3 activation, and possibly also affect the degradation of c-Met protein, similar to its effect on EGFR. c-Met, on the other hand, enhances the phosphorylation of PYK2 and STAT3 ( Fig. 9c and Supplementary Fig. 6 ) and also the expression of EMT transcription factors ( Fig. 9d ). These observations suggest that a positive feedback in the PYK2–STAT3–c-Met axis contributes to EMT in breast cancer ( Fig. 9e ), and that disruption of this axis might be an effective therapeutic approach for certain breast cancer subtypes. Consistent with this hypothesis, previous studies suggest that the c-Met inhibitor PHA-665752 synergizes with the EGFR inhibitor erlotinib to decrease the viability of MDA-MB-468 cells, and that the combination of EGFR and c-Met inhibitors could be effective treatment for triple-negative breast cancer patients [62] . Given that PYK2 is a common downstream effector of EGFR ( Fig. 5a ) and c-Met ( Supplementary Fig. 6d ), it could be that PYK2 inhibitor would effectively reduce the progression and metastasis of specific breast cancer subtype or might synergize with inhibitors for c-Met or EGFR. Further studies are required to explore this possibility. In summary, we describe here a signalling network between EGFR, c-Met, PYK2 and STAT3 ( Fig. 9e ), and demonstrate how the crosstalk and interplay between these signalling components prolong signal duration and potentiate EMT. The profound effect of PYK2 on EMT, and the significant correlation between PYK2 expression, high-grade tumours and LNM in human breast cancer patients ( Fig. 4 ) emphasizes the clinicopathological implication of the current findings. Antibodies reagents and chemicals Monoclonal anti-HA antibody and rabbit polyclonal antibodies against pPYK2 (Y402) (sc-101790, 1:1,000 WB, 1:200 IF), STAT3 (C-20, 1:1,000)), FAK (sc-558, 1:1,000), ERK1/2 (sc-93, 1:1,000), pERK1/2(sc-136521, 1:500), AKT (sc-8312, 1:1,000), E-cadherin (sc-8426, 1:1,000 WB, 1:200 IF), LAMP3 (sc-15363; IF 1:300) and α-Tubulin (sc-9104, 1:1,000) were purchased from Santa Cruz Biotechnology (Santa Cruz, CA). Rabbit polyclonal antibody against PYK2 used in IH was from Sigma. Antibodies against pAKT (T308, #2965 and S473, #9271, 1:1,000), pSTAT3 (Y705, #9145, 1:1,000 WB, 1:200 IF), pc-Met (Y1234/5, #3077, 1:1,000), pFAK (Y397, #8556, 1:1,000), pSrc (Y416, #6943, 1:1,000 WB, 1:100 IF) and c-Met (#8198, 1:1,000 WB, 1:100 IF) were purchased from Cell Signaling Technologies (Beverly, MA). Antibodies against fibronectin (HFN7.1c, 1:500), CD44 (H4C4-c, 1:500) and vimentin (AMF-17b, 1:500) were purchased from Developmental Studies Hybridoma Bank (Iowa City, IA). Monoclonal anti-EEA1 antibody (ab70521, IF 1:1,000) and p38MAPK (ab32557, 1:1,000) was purchased from Abcam (Cambridge, MA), while monoclonal anti-EGFR antibody (clone 111.6, 1:5,000 WB, 1:1,000 IF) was kindly provided by Professor Y. Yarden (Weizmann Institute of Science, Rehovot, Israel). Polyclonal anti-PYK2 antibody was prepared as described previously [25] . Alexa-488 donkey anti-mouse and anti-rabbit IgGs were purchased from Invitrogen (Carlsbad, CA). Cyanine (Cy)3-conjugated goat anti-rabbit and goat anti-mouse IgGs were purchased from Jackson ImmunoResearch Laboratories (West Grove, PA). AG490, Stattic, S31-201 and PP2 were purchased from Calbiochem. TGFβ and HGF were purchased from ProSpec (Israel). EGF, Hoechst 33342, PHA-665752 and other chemicals were purchased from Sigma. Cell culture and immunofluorescence analysis MCF10A, MDA-MB-468, BT-549, BT-20 and Human embryonic kidney (HEK-293T) cells were obtained from ATCC. MCF10A cells were grown in DMEM:F12 (1:1) medium supplemented with EGF (10 ng ml −1 ), Insulin (10 μg ml −1 ), Cholera Toxin (1 μg ml −1 ), Hydrocortisone (1 μg ml −1 ) and heat-inactivated horse serum (5%). MDA-MB-468 and BT-549 cells were grown in RPMI (Gibco BRL; Grand Island, NY) medium supplemented with 10% fetal calf serum (FCS). Insulin (0.023 IU ml −1 ) was added to the growth media of BT-549 cells. BT-20 cells were grown in Eagle’s Minimum Essential Medium (MEM-Eagle’s) supplemented with 10% FCS, 2 mM L -glutamine and 1 mM sodium pyruvate. HEK-293T cells were grown in DMEM (Gibco BRL; Grand Island, NY) supplemented with 10% heat-inactivated fetal bovine serum (Gibco BRL, Grand Island, NY), 1 mM sodium pyruvate and a penicillin–streptomycin mixture (100 U ml −1 ; 0.1 mg ml −1 ; Beit Haemek, Israel). Immunofluorescence analysis was performed essentially as described previously [63] . In brief, the cells were grown on coverslips, treated with EGF as indicated and then washed with PBS and fixed with 4% paraformaldehyde (PFA) in PBS for 20 min at room temperature. The fixed cells were incubated for 15 min in PBS containing 0.1 M glycine, followed by 30 min incubation in blocking buffer (10 mM Tris, pH 7.5, 150 mM NaCl, 10% goat serum, 2% bovine serum albumin in Tris-buffered saline and 0.1% Triton-X-100) and then by 1 h incubation with the indicated primary antibodies diluted in the blocking buffer. The cells were then washed with PBS and incubated for 1 h with fluorescence-labelled secondary antibodies. After washing with PBS, the cells were incubated for 5 min with 2 ng μl −1 Hoechst 33342, washed again with PBS and mounted on microscopic slides using mounting media (10 mM phosphate buffer, pH 8.0, 16.6% w/v Mowiol 4–88 and 33% glycerol). The specimens were analysed by a confocal laser-scanning microscope (LSM 510; Carl Zeiss) equipped with a 63 Å/1.4 oil differential interference contrast M27 objective lens (Plan Apochromat; Carl Zeiss) using the 488-, 543- and either 405- or 633-nm excitation for fluorescein, Cy3 epifluorescence and either 4,6-diamidino-2-phenylindole (Hoechst) or Cy5, respectively. Images were acquired using the LSM 510 software. Co-localization analysis Co-localization was measured using the Zeiss LSM 510 meta software, essentially as previously described [64] . In brief, the overlapping regions between the green and red channels, which appeared in yellow in the merged confocal images, were marked as regions of interest in randomly selected cells ( n >20). To generate the scatter plots, all pixels above the background (which is automatically calculated by the software at the mean fluorescence intensity) in the red and green channels were considered. The relative numbers of red pixels co-localized with the green pixels were compared with the total number of both red and green pixels and Manders’ co-localization coefficient [65] was calculated by the software. The co-localization coefficient ranges between no co-localization (0) and complete co-localization (1) of red and green pixels. Data were expressed in mean (±s.d.) of three different experiments and statistical significance of co-localization was evaluated with the Student’s t -test. DNA constructs and lentivirus production and infection Two different shRNA sequences were used to downregulate PYK2 expression. The first one (No.1) was purchased from Sigma (TRCN00000231519), whereas the second one (No. 2) was described previously [66] . The PYK2 shRNAs were cloned into the pLKO.1-puro lentiviral vector. HA-tagged wild-type PYK2 was subcloned into the pHAGE PGK-IRES-Hygro-W lentiviral vector. Lentivirus production and infection were conducted essentially as described previously [63] , [67] . EMT induction and WB analysis To induce EMT in MCF10A cells, the cells were grown in the absence of EGF for 24 h and then stimulated with EGF (10 ng ml −1 ) or TGF-β (5 ng ml −1 ) for 5 days. To induce EMT in MDA-MB-468 cells, the cells were serum starved (0.5% FCS) for 24 h and then stimulated with EGF (50–100 ng ml −1 ) for 24–72 h. EMT transcription factors were assessed after 24 h (RT–PCR) and cellular protein markers were examined after 72 h (WB). Cells were extracted in lysis buffer (0.1% Triton-X-100, 50 mM Hepes pH 7.5, 100 mM NaCl, 1 mM MgCl 2 , 50 mM NaF, 0.5 mM NaVO 3 , 20 mM β-glycerophosphate, 1 mM phenylmethylsulphonyl fluoride, 10 μg ml −1 leupeptin, 10 μg ml −1 aprotinin). Cell lysates were centrifuged at 14,000 r.p.m. for 15 min at 4 °C. Protein concentration of the supernatants was determined by Bradford assay (Bio-Rad, Hercules, CA) and equal protein amounts (60–80 μg) were analysed by SDS–polyacrylamide gel electrophoresis and WB. Densitometric analysis was performed using the ImageJ software (NIH, USA). Uncropped scans of WB are available in Supplementary Figs 8 to 18 . RNA extraction and RT–PCR RNA was purified using the TRI Reagent (Sigma). RNA (2 μg) was reverse transcribed using the SuperScriptII first strand synthesis kit (Invitrogen). RT–PCR was performed using Red-taq mix (Sigma-Aldrich, Israel). For real-time PCR analysis, SYBR Green I was used as a fluorescent dye and amplifications were performed according the manufacturer’s guidelines (Invitrogen) using the ABI StepOnePlus 7500 Real-time PCR system (Perkin-Elmer Applied Biosystems). Real-time PCR primers were designed using the Primerexpress software of Applied Biosystems (Invitrogen). The oligonucleotide primers used in these studies are listed in Supplementary Table 1 . All experiments were carried out in triplicates and normalized to actin RNA levels. Cell migration and invasion MDA-MB-468 cells (10 5 cells per insert) were plated in the upper compartment of a Transwell tray (BD Bioscience, San Jose, California). The bottom of the insert was coated with 10 μg ml −1 Fibronectin for 2 h before cell plating. The cells were incubated in serum-free medium for 16 h and allowed to migrate through the intervening polycarbonate membrane (8-μm pore size) toward EGF (50 ng ml −1 ) in the lower chamber. Thereafter, the inserts were gently removed and washed with PBS. The cells on the upper surface of the filter were removed, and the migrated cells on the bottom side of the filter were fixed in saline containing PFA (3%), permeabilized in Triton-X-100 (0.05%) and stained with methyl violet (0.02%). Microscopic images were captured to visualize the migrated cells. Cells were counted in five fields of triplicate membranes and the results were plotted as fold of control. For cell invasion assays, 10 5 cells per insert (MDA-MB-231) or 5 × 10 4 cells per insert (BT-549) were plated in the upper compartment of BioCoat Matrigel Chambers (BD Bioscience, San Jose, California) in a serum-free media. The cells were allowed to invade towards EGF (50 ng ml −1 ) in the lower chamber for 16 h and processed as above. Wound-healing assays were performed according to the manufacturer’s protocol (iBidi, Germany). In brief, the cells were trypsinized and diluted in normal medium at 10 6 cells ml −1 and 70 μl were plated into each well, resulting in a confluent layer within 16 h. Thereafter, the insert was removed and cells were allowed to migrate for different time points. The experiments were done in the presence of 10 μM mitomycin C to inhibit cell proliferation. Percentage of wound closure was determined by measuring the gap between the wounded monolayers. Chromatin immunoprecipitation ChIP was performed as descried previously [60] with some modifications. In brief, MDA-MB-468 cells (10 7 ) were serum starved (0.5% serum) for 24 h and then stimulated with EGF (100 ng ml −1 ) for 30 min. The cells were incubated in 1% PFA for 10 min at room temperature to crosslink and stabilize protein–DNA complexes. The cells were then washed with PBS/0.125 M glycine for 5 min and extracted in 800 μl RIPA buffer (10 mM Tris-HCl pH 8.0, 1 mM EDTA pH 8.0, 140 mM NaCl, 1% Triton-X-100, 0.1% SDS, 0.1% DOC, 1 μg ml −1 aprotinin and 1 mM phenylmethylsulphonyl fluoride). Cell extracts were incubated on ice for 10 min and sonicated using Branson 250 Sonifier sonicator (Emerson Electric Co., MO, USA) to sheer chromatin and DNA into ~500–300 bp DNA fragments. The sonicated lysates were centrifuged at 14,000 r.p.m. for 15 min at 4 °C, and the supernatants were precleared with normal IgG bound to protein A-agarose beads. The samples were then immunoprecipitated with either anti-STAT3 antibody or normal IgG for 12 h at 4 °C. The immunocomplexes were then incubated with 6 μg salmon sperm DNA for 1 h at 4 °C. Immunoprecipitates were washed twice with cold RIPA buffer, twice with cold LiCl buffer (10 mM Tris-HCl pH 8.0, 1 mM EDTA pH 8.0, 250 mM LiCl, 0.5% NP-40, 0.5% DOC) and finally with cold TE buffer (10 mM Tris-HCl pH 8.0, 1 mM EDTA pH 8.0). DNA–protein complexes were eluted using 50 μl elution buffer (10 mM Tris-HCl pH 8.0, 5 mM EDTA pH 8.0, 300 mM NaCl and 0.5% SDS) and incubated with RNase A (0.2 mg ml −1 ) for 30 min at 37 °C. The crosslinked DNA–protein complexes were then dissociated by incubating the samples at 65 °C for 16 h. The DNA was purified utilizing a PCR purification kit (Promega) and amplified by PCR using specific oligonucleotide primers ( Supplementary Table 4 ). Immunohistochemistry Anonymized tissue samples of invasive breast cancer cases were collected from patients undergoing surgical resection at the Department of Gynecology and Obstetrics at the Goethe University in Frankfurt, Germany. The tissue samples were obtained with the institutional review board approval (Ethik-Kommission Fachbereich Medizin der Goethe-Universität Frankfurt) and patient’s written informed consent. Samples were characterized according to standard pathology including oestrogen receptor, progesterone receptor and HER2 status. IH was performed as described previously [68] on 3-μm serial sections from formalin-fixed, paraffin-embedded breast carcinoma. In brief, the sections were deparaffinized by 10-min incubation at 60 °C followed by 15-min immersion in xylene. The sections were then rehydrated by sequential incubation in 100, 96 and 70% ethanol (10 min each). Samples were rinsed with PBS (3 min) followed by distilled water (2 × 3 min) and then incubated for 30 min in methanol/H 2 0 2 (0.9%) solution to quench endogenous peroxidases. The sections were incubated in Tris-EDTA buffer (10 mM Tris-HCl, 1 mM EDTA, pH 9.0) and antigen retrieval was performed by microwave irradiation for 10 min. Samples were then incubated for 1 h in blocking buffer containing 20% normal horse serum and 0.2% Triton-X-100 in PBS, and then with rabbit anti-PYK2 antibody (P3902, 1:50, Sigma-Aldrich) for 12–16 h at room temperature. Thereafter, the slides were washed three times (15 min each) in PBS and then incubated for 1.5 h with biotinylated donkey anti-rabbit antiserum (DakoCytomation; 1:100) followed by 2 h incubation with StreptABComplex/HRP (DakoCytomation; according to the manufacturer’s protocol). The samples were washed with 0.1 M phosphate buffer and antibody binding was assessed by monitoring HRP activity using diaminobenzidine staining solution (0.2 mg ml −1 diaminobenzidine, 0.01% H 2 0 2 in 0.1 M phosphate buffer). Negative controls were treated similarly without primary antibody. Sections were then counterstained with haematoxylin and eosin, dehydrated and mounted on coverslips. Scoring of tissue samples Samples from 92 breast cancer patients and 10 normal breast tissues were stained. The intensity of specific staining was characterized as negative (0), low (1+), moderate (2+) and high (3+). For each sample, H-Score was calculated as described elsewhere [68] . Tumour grade was evaluated according to clinical and pathological data. Statistics were performed using χ 2 -analysis. Luciferase assay Amplified PCR fragments containing the putative STAT3-binding sites (Sequence 1, 2) were subcloned into the pGL2 luciferase reporter vector (Promega) upstream to the luciferase gene. The plasmids were expressed together with a β-Galactosidase reporter plasmid (pSV-β-Galactosidase, Promega) in MDA-MB-468 cells. Twenty-four hours after transfection (LipofectAMINE 2000, Invitrogen), the cells were serum starved for 12 h and then stimulated with EGF (100 ng ml −1 ) for 4 h in the presence or absence of Stattic (10 μM), S31-201 (300 μM) or AG490 (100 μM). The cells were then lysed and luciferase activity was measured using the dual-light luciferase and β-Galactosidase reporter gene assay system (Promega) according to the manufacturer’s instructions. Results were normalized with β-Galactosidase activity and plotted as relative luciferase activity with respect to the empty vector (pGL2) control. How to cite this article : Verma, N. et al . PYK2 sustains endosomal-derived receptor signalling and enhances epithelial-to-mesenchymal transition. Nat. Commun. 6:6064 doi: 10.1038/ncomms7064 (2015).